NK1.1+CD8+T cells escape TGF-β control and contribute to early microbial pathogen response Following microbial pathogen invasion, one of the main challenges for the host is to rapidly control pathogen spreading to avoid vital tissue damage. Here we report that an effector CD8 + T-cell population that expresses the marker NK1.1 undergoes delayed contraction and sustains early anti-microbial protection. NK1.1 + CD8 + T cells are derived from CD8 + T cells during priming, and their differentiation is inhibited by transforming growth factor-β signalling. After their own contraction phase, they form a distinct pool of KLRG1 CD127 double-positive memory T cells and rapidly produce both interferon-γ and granzyme B, providing significant pathogen protection in an antigen-independent manner within only a few hours. Thus, by prolonging the CD8 + T-cell response at the effector stage and by expressing exacerbated innate-like features at the memory stage, NK1.1 + cells represent a distinct subset of CD8 + T cell that contributes to the early control of microbial pathogen re-infections. CD8 + T cells have been largely depicted as potent effector lymphocytes in the eradication of numerous intracellular pathogens including bacteria and viruses. During CD8 + T-cell response to an acute infection, naïve CD8 + T cells, carrying an appropriate T-cell receptor (TCR), specifically recognize pathogen-derived antigens presented by major histocompatibility complex (MHC)-I to undergo an activation-phase characterized by a vigorous proliferative burst, resulting in the formation of a large pool of effector T cells. This expansion is associated with the acquisition of effector functions. A large proportion of CD8 + T cells acquire cytotoxic molecules and effector cytokines (interferon (IFN)-γ, tumour necrosis factor (TNF)-α) and the capacity to kill infected cells as well as to recruit or activate other cells of the immune system, resulting in effective pathogen clearance [1] , [2] . The CD8 response typically peaks around 6–7 days after infection, and 90–95% of the effector T cells are then destroyed in the following days and weeks by apoptosis, whether the pathogen is totally eliminated or not [3] . The fraction of effector cells surviving this contraction-phase will persist long term in an antigen-independent manner in mice and humans [4] . These memory cells can blunt the severity of a second infection, by proliferating and producing cytokines quickly after pathogen infection [1] . However, it has been reported that at the peak of expansion following certain infections or immunizations, a small fraction of cells exhibit features of memory antigen-specific cells [5] , [6] . Their potential to proliferate and acquire effector function appears to be blocked by the presence of effector cells [6] , and it takes approximately 40 days for these cells to acquire full memory cell qualities [7] . Moreover, a few days are required to establish an efficient antigen-specific response by memory CD8 + T cells following a secondary microbial infection [8] . Thus, the death of antigen-specific effector cells in the contraction phase delays the re-establishment of a fully effective arsenal of CD8 + T cells, and could lead to early pathogen propagation upon rapid re-infection. Conversely, recent observations revealed a heterogeneity at the initiation of the contraction phase depending on the priming conditions, suggesting that some effector CD8 + T cells could prolong protection because of their delayed contraction [9] , [10] . Moreover, at the memory stage, we and others have reported that pathogen-specific CD8 + T cells can respond to inflammatory cytokines by producing both IFN-γ and granzyme B in an antigen-independent manner within a few hours following pathogen entry [11] , [12] , [13] , [14] , [15] . Thus, in order to improve microbial pathogen protection, it is essential to identify CD8 + T cell subsets that can either contract later and/or respond earlier to second infections, as well as to determine factors controlling their differentiation. During the last decade, it has become clear that antigen-induced effector CD8 + T cells are phenotypically heterogeneous [16] . At the peak of the response, cells harbouring IL-7Rα (CD127) and lacking the killer cell lectin-like receptor G1 (KLRG1) were reported to survive the contraction phase and give rise to memory cells, whereas KLRG1-positive cells were regarded as short-lived effector cells [1] . Interestingly, other markers usually associated with NK cells have also been observed on some CD8 + T lymphocytes. Among them, the glycoprotein NK1.1 was reported at the surface of some CD8 + T cells during viral infections in both mice and humans [17] , [18] , [19] . Although NK1.1 + CD8 + T cells have been described for more than a decade, their contribution in the CD8 response against microbial infection, as well as the factors controlling their differentiation in vivo, remains elusive. We show that, upon viral or bacterial infections in mice, a fraction of CD8 + T cells can escape transforming growth factor-β (TGF-β) control during priming, giving rise to NK1.1 + CD8 + T cells. These TGF-β-repressed CD8 + T cells represent a unique pathogen-specific subset. In contrast to their NK1.1 − counterparts, NK1.1 + CD8 + T cells undergo delayed contraction, and provide prolonged pathogen-specific reactivity to the host. The fraction of NK1.1 + CD8 + T cells that survives the contraction phase maintains KLRG1 surface expression. These memory cells rapidly produce both IFN-γ and granzyme B, not only in response to pathogen antigens, but also in an antigen-independent manner, providing an early protection against invading microbial pathogens. Overall, our results reveal both the origin and the function of NK1.1 + CD8 + T cells, a key subset of T lymphocytes that sustains early CD8 + T cell-mediated host protection against microbial pathogen re-infections. NK1.1 + CD8 + T-cell differentiation is repressed by TGF-β signalling CD8 + T-cell heterogeneity is believed to be largely influenced by factors controlling the initial priming during microbial infection [20] , [21] . Among the factors able to influence the differentiation of numerous T-cell subsets, cytokines, and particularly TGF-β, are regarded as potent actors [22] . This pleiotropic cytokine signals through a two-receptor complex composed of TGF-βRI and TGF-βRII. Signalling is initiated by the auto-phosphorylation of the TGF-βRII subunit, which in turn phosphorylates TGF-βRI, activating several signalling pathways [23] . First, we sought to examine whether microbial infections affected sensitivity of T lymphocytes to TGF-β. Wild-type C57BL/6 (B6) mice were infected with lymphocytic choriomingitis virus Armstrong strain (LCMV), and TGF-βRII expression was analysed at the surface of T cells 8 days later. Strikingly, infection was associated with a loss of expression of TGF-βRII at the surface of around half of CD8 + T cells ( Fig. 1a ). This feature was confined to CD8 + T cells, as surface TGF-βRII expression remained almost stable on CD4 + T cells. Interestingly, in clear contrast with cells that maintained high levels of TGF-βRII expression, we found that the TGF-βRII low CD8 + population was enriched in T cells expressing the glycoprotein NK1.1 ( Fig. 1a ), whereas activated T lymphocytes, based on CD44, CD62L and Ly6C expression, were almost equally distributed between TGF-βRII low and TGF-βRII high populations after LCMV infection ( Supplementary Fig. 1a ). After infection, NK1.1 + CD8 + T cells were mainly observed within the spleen, the blood and the liver, but were barely detectable in the lymph nodes and not found in the thymus ( Supplementary Fig. 1b ). Notably, in addition to NK1.1, we found that TGFβRII low CD8 + T cells also expressed high levels of various surface receptors characteristic of NK cells, including DX5, CD94, NKG2A/C/E, NKG2D and LY49C/I/F ( Supplementary Fig. 1c ). Moreover, NK1.1 + CD8 + T cells generated in response to LCMV, exhibited a diverse α,β TCR repertoire and their development was not impaired in CD1d KO LCMV-infected mice, ruling out a potential NKT cell lineage origin for these cells ( Supplementary Fig. 1d-e ). The low levels of TGF-βRII at the surface of NK1.1 + CD8 + T cells suggested that TGF-β signalling could repress the development of these cells. To verify this, we created mixed bone marrow (BM) chimera mice by reconstituting sub-lethally irradiated Rag-deficient mice (RAG KO ) with BM (ratio 1:1) from both Thy1.1 B6 mice and Thy1.2 CD4-cre; LsL TgfbRI CA B6 (TGFβ-RI CA ) mice. The latter express a constitutively active form of TGF-βRI selectively in their αβ T cells [24] . In response to LCMV infection, we observed that very few NK1.1 + CD8 + T cells were derived from TGFβRI CA BM, whereas NK1.1 − CD8 + T cells were equally provided by both TGFβRI CA BM and TGFβRI WT BM ( Fig. 1b,c ) demonstrating the repressive effect of TGF-β on NK1.1 + CD8 + T-cell differentiation. To follow the kinetics of NK1.1 + CD8 + T-cell appearance, we analysed LCMV peptide-MHC-tetramer-positive CD8 + T cells from day 2 to the peak of the response at day 8. In line with a decreasing sensitivity to TGF-β because of a gradual loss of TGF-βRII at the surface of CD8 + T cells from day 5 ( Fig. 1d ), significant numbers of NK1.1 + CD8 + T cells were only detected after the fifth day of LCMV infection ( Fig. 1e ). It was notable that, like their NK1.1 − counterparts, NK1.1 + CD8 + T cells specific for LCMV antigen gradually acquired KLRG1 at their surface, ( Supplementary Fig. 2a,b ), refuting the possibility that they are derived from KLRG1 + effector cells. Moreover, NK1.1 + CD8 + T-cell differentiation was also observed in the spleen of mice grafted with purified naïve NK1.1 − CD8 + T cells from ovalbumin peptide (Ova)-specific OT-1 TCR transgenic mice and infected with Listeria monocytogenes bacteria expressing Ova ( Lm- Ova), ruling out a viral infection-restricted effect and suggesting a differentiation of NK1.1 + CD8 + T cells in response to microbial pathogen infection during priming of naïve NK1.1 − CD8 + T cells before KLRG1 expression ( Fig. 1f,g ). Thus, this first set of data reveal that TGF-β directly influences the heterogeneity of the CD8 + T-cell population by repressing the differentiation of NK1.1 + CD8 + T cells from NK1.1 − CD8 + T cells during microbial pathogen infections. 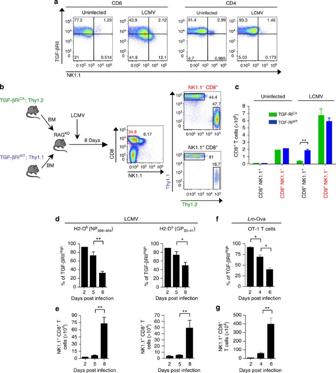Figure 1: TGF-β signalling represses NK1.1+CD8+T-cell differentiation. (a) Flow cytometry analysis of TGF-βRII and NK1.1 expression at the surface of either CD8+T-cell splenocytes or CD4+T-cell splenocytes 8 days after LCMV infection of B6 mice. Data are representative of four experiments with three or four animals per group. (b,c) T cell-depleted bone marrow (BM) cells fromCD4-Cre; Stopfl/flTgf-βRICAThy1.2 B6 mice (TGF-βRICA) or Thy1.1 B6 mice (TGF-βRIWT) were mixed at a 1:1 ratio and transferred into irradiatedrag2KOmice (RAGKO). Chimeras were infected with LCMV 5 weeks later and splenocytes analysed by flow cytometry 8 days post infection for the BM origin of NK1.1+CD8+T splenocytes. (c) Graph illustrating the absolute number of NK1.1+CD8+T cells and NK1.1−CD8+T splenocytes derived from each BM donor (mean+s.d.,n=3 representative of 2 experiments). (d) Graph illustrating the percentage of both LCMV-specific H2-Db(NP396–404) tetramer+CD8+splenocytes and LCMV-specific H2-Db(GP33–41) tetramer+CD8+splenocytes expressing high levels of TGF-βRII at different times after LCMV infection. (e) Graph illustrating absolute numbers of LCMV-specific H2-Db(NP396–404) and LCMV-specific H2-Db(GP33–41) tetramer+CD8+splenocytes expressing NK1.1 at different times after LCMV infection. Data are representative of three experiments and shown as mean+s.d.n=5 per point. (f,g) Naïve (CD44lowCD62Lhigh) OT-1 T cells were adoptively transferred into B6 mice, infected the following day byLm-Ova.The graphs illustrate the percentage of OT-1 splenocytes expressing high levels of TGF-βRII (f) and the absolute numbers of NK1.1+OT-1 T cells at different times afterLm-Ova infection (g). Data are representative of three experiments and shown as mean+s.d.n=3 per point. Unpaired, two-tailed Student’st-test was used to assess the significance of differences observed between two groups.*P<0.05; **P<0.001. Figure 1: TGF-β signalling represses NK1.1 + CD8 + T-cell differentiation. ( a ) Flow cytometry analysis of TGF-βRII and NK1.1 expression at the surface of either CD8 + T-cell splenocytes or CD4 + T-cell splenocytes 8 days after LCMV infection of B6 mice. Data are representative of four experiments with three or four animals per group. ( b , c ) T cell-depleted bone marrow (BM) cells from CD4-Cre; Stop fl/fl Tgf- β RI CA Thy1.2 B6 mice (TGF-βRI CA ) or Thy1.1 B6 mice (TGF-βRI WT ) were mixed at a 1:1 ratio and transferred into irradiated rag2 KO mice (RAG KO ). Chimeras were infected with LCMV 5 weeks later and splenocytes analysed by flow cytometry 8 days post infection for the BM origin of NK1.1 + CD8 + T splenocytes. ( c ) Graph illustrating the absolute number of NK1.1 + CD8 + T cells and NK1.1 − CD8 + T splenocytes derived from each BM donor (mean+s.d., n =3 representative of 2 experiments). ( d ) Graph illustrating the percentage of both LCMV-specific H2-D b (NP 396–404 ) tetramer + CD8 + splenocytes and LCMV-specific H2-D b (GP 33–41 ) tetramer + CD8 + splenocytes expressing high levels of TGF-βRII at different times after LCMV infection. ( e ) Graph illustrating absolute numbers of LCMV-specific H2-D b (NP 396–404 ) and LCMV-specific H2-D b (GP 33–41 ) tetramer + CD8 + splenocytes expressing NK1.1 at different times after LCMV infection. Data are representative of three experiments and shown as mean+s.d. n =5 per point. ( f , g ) Naïve (CD44 low CD62L high ) OT-1 T cells were adoptively transferred into B6 mice, infected the following day by Lm-Ova. The graphs illustrate the percentage of OT-1 splenocytes expressing high levels of TGF-βRII ( f ) and the absolute numbers of NK1.1 + OT-1 T cells at different times after Lm- Ova infection ( g ). Data are representative of three experiments and shown as mean+s.d. n =3 per point. Unpaired, two-tailed Student’s t -test was used to assess the significance of differences observed between two groups. *P <0.05; ** P <0.001. Full size image Dual role for IL-15 and TGF-β in NK1.1 + CD8 + T-cell differentiation Because inflammatory conditions during CD8 + T-cell priming are known to influence the heterogeneity of the CD8 + T cells [20] , [21] , we next investigated whether pro-inflammatory factors associated with microbial infection promote NK1.1 + CD8 + T-cell differentiation. As IL-15 levels can increase in response to infections [25] , [26] , and IL-15 signalling has been proposed to repress of TGF-β signalling on cultured CD8 + T lymphocytes [27] , we further assessed the contribution of IL-15 to NK1.1 + CD8 + T-cell differentiation in vivo . For this, Il-15 competent (IL-15 WT ) or Il-15- deficient (IL-15 KO ) B6 mice were grafted with OT-1 cells and subsequently infected with Lm -Ova ( Fig. 2a–d ). Taking into consideration that IL-15 is critical for CD8 + T-cell homeostasis [28] , splenocytes were analysed at day 6 after infection when the proportion of OT-1 KLRG1 + effector cells remained similar between il-15 wt and il-15 KO mice. However, in the absence of IL-15, we observed a 50% reduction of NK1.1 + OT-1 cells, revealing a positive role for IL-15 on NK1.1 + CD8 + T-cell differentiation ( Fig. 2d ). Moreover, TGF-βRII expression at the surface of OT-1 cells remained relatively high in il-15 KO mice compared with that of grafted il-15 wt animals, strongly suggesting that IL-15 signalling decreased the sensitivity of CD8 + T cells to TGF-β ( Fig. 2b–d ). Interestingly, in both IL-15-deficient and -sufficient mice, the levels of TGF-βRII at the surface endogenous of T cells remained higher than that of OT-1 cells. In addition, endogenous T cells failed to differentiate efficiently in NK1.1 + CD8 + T cells ( Fig. 2b ) implying that, in addition to cytokines produced during infection, such as IL-15, TCR engagement might also be required to enhance NK1.1 + CD8 + T-cell differentiation. Altogether, these data revealed that, during infection, the differentiation of NK1.1 − CD8 + T cells into NK1.1 + CD8 + T cells is influenced by a dual role of TGF-β and IL-15 during TCR priming. IL-15 facilitates TGF-β receptor downregulation on CD8 + T cells, and their differentiation in NK1.1 + cells. 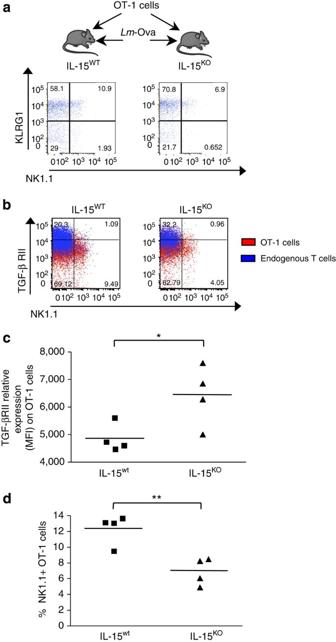Figure 2: TGF-β and IL-15 play a dual role in NK1.1+CD8+T-cell differentiation. (a–d) Tomato+OT-1 CD8+T cells were transferred into either IL-15-deficient mice or IL-15-sufficient B6 mice infected the following day withLm-Ova. (a) Flow cytometry analysis of the co-expression of NK1.1 and KLRG1 at the surface of OT-1 cells 6 days after infection. (b) Flow cytometry analysis of the co-expression of NK1.1 and TGF-βRII at the surface of either transferred or endogenous CD8+T cells 6 days after infection. Quadrant digits indicate the proportion of cells expressing NK1.1 and TGF-βRII among the total CD8+T splenocytes. (c,d) Graphs illustrate the proportion of NK1.1+cells among CD8+T splenocytes as well the mean of fluorescence intensity (MFI). These results are representative of two independent experiments with four or five recipient mice per group. Unpaired, two-tailed Student’st-test was used to assess the significance of differences observed between two groups.*P<0.05; **P<0.001. Figure 2: TGF-β and IL-15 play a dual role in NK1.1 + CD8 + T-cell differentiation. ( a – d ) Tomato + OT-1 CD8 + T cells were transferred into either IL-15-deficient mice or IL-15-sufficient B6 mice infected the following day with Lm -Ova. ( a ) Flow cytometry analysis of the co-expression of NK1.1 and KLRG1 at the surface of OT-1 cells 6 days after infection. ( b ) Flow cytometry analysis of the co-expression of NK1.1 and TGF-βRII at the surface of either transferred or endogenous CD8 + T cells 6 days after infection. Quadrant digits indicate the proportion of cells expressing NK1.1 and TGF-βRII among the total CD8 + T splenocytes. ( c , d ) Graphs illustrate the proportion of NK1.1 + cells among CD8 + T splenocytes as well the mean of fluorescence intensity (MFI). These results are representative of two independent experiments with four or five recipient mice per group. Unpaired, two-tailed Student’s t -test was used to assess the significance of differences observed between two groups. *P <0.05; ** P <0.001. Full size image NK1.1 + CD8 + T lymphocytes are potent effector cells It is well established that after recognition of pathogen antigens, CD8 + T cells undergo an activation-phase characterized by a vigorous proliferative burst in the first week of infection, resulting in the formation of a large pool of cells producing effector cytokines. We next assessed whether NK1.1 + CD8 + T cells were endowed with similar features in response to infectious agents. Using LCMV-specific tetramers, we first compared NK1.1 + CD8 + and NK1.1 − CD8 + T-cell clonal expansion by giving drinking water containing 5-bromodeoxyuridine (BrdU) to mice during the first 8 days following LCMV injection. We observed a modest, although not significant, increased proportion of BrdU + among the NK1.1 + CD8 + T cells at day 5 after infection as compared with NK1.1 − CD8 + T cells. The upregulation of CD44 and the downregulation of CD62L, commonly used to monitor T-cell activation, was similar between NK1.1 + and NK1.1 − LCMV-specific CD8 + T cells, both at days 5 and 10 after infection ( Supplementary Fig. 3a,b ). However, we found that LCMV-specific NK1.1 + CD8 + T cells were mainly KLRG1 positive 10 days after LCMV infection as compared with NK1.1 − CD8 + T cells ( Fig. 3a,b ). Moreover, in clear contrast to their NK1.1 − counterparts, NK1.1 + KLRG1 + CD8 + T cells massively expressed both IFN-γ and TNF-α ex-vivo in response to LCMV peptide stimulation ( Fig. 3a,b ). 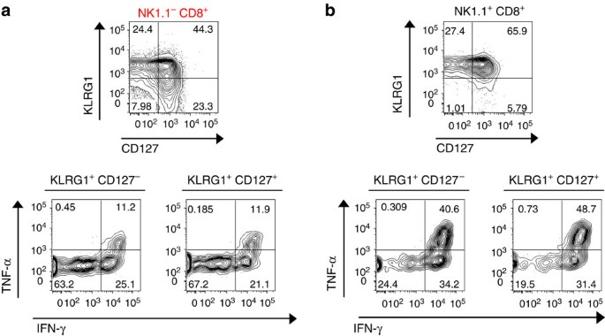Figure 3: NK1.1+CD8+T cells consist of activated and effector cells. (a,b) B6 mice were infected with LCMV and their spleens analysed 9 days later by flow cytometry. Expression of surface expression of KLRG1 and CD127 as well as IFN-γ and TNF-α production by H2-Db(NP396–404) tetramer+CD8+T cells after 3 h of culture with LCMV NP396peptide-pulsed antigen-presenting cell. These results are representative of two independent experiments with three mice per group. Notably, we did not find significant difference in granzyme B production between the two subsets, however, a large proportion of NK1.1 + KLRG1 + CD8 + T cells expressed the degranulation associated molecule Lamp1 (CD107) at their surface compared with NK1.1 − KLRG1 + CD8 + T cells ( Supplementary Figure 3b ). Thus, these data reveal that, in response to infection, NK1.1 + CD8 + T cells represent a potent effector CD8 + T-cell population, and support the use of NK1.1 as a surface marker to discriminate CD8 + T cells with exacerbated effector functions. Figure 3: NK1.1 + CD8 + T cells consist of activated and effector cells. ( a , b ) B6 mice were infected with LCMV and their spleens analysed 9 days later by flow cytometry. Expression of surface expression of KLRG1 and CD127 as well as IFN-γ and TNF-α production by H2-D b (NP 396–404 ) tetramer + CD8 + T cells after 3 h of culture with LCMV NP 396 peptide-pulsed antigen-presenting cell. These results are representative of two independent experiments with three mice per group. Full size image NK1.1 + CD8 + T lymphocytes are long-lived effector cells The activation and expansion of effector cells are usually followed by a drastic reduction in their number due to large-scale apoptotic death [2] . We then monitored the numbers of NK1.1 + CD8 + T cells and NK1.1 − CD8 + T cells specific for a same LCMV immunogenic peptide at different time points post infection ( Fig. 4a ). Surprisingly, although 60–70% of NK1.1 − CD8 + T cells were lost between day 8 and 21 post infection ( Fig. 4a,b ), the population size of NK1.1 + CD8 + T cells specific for the same LCMV peptide remained almost constant until the fourth week following infection, whereupon it started to significantly decrease. As a consequence of this delayed contraction, NK1.1 + CD8 + T lymphocytes, which represented only 10–15% of LCMV-specific CD8 + T cells at day 10, represented 40–60% of LCMV-specific CD8 + T cells at day 28, before returning to around 10% by day 60 ( Fig. 4c,d ). Moreover, 3 weeks after infection, twice more NK.1.1 + CD8 + T cells maintained the effector phenotype KLRG1 + CD127 − compared with their NK1.1- counterparts ( Fig. 4e ). This delayed contraction suggests that NK1.1 + CD8 + T cells could be more resistant than their CD8 + T-cell counterparts to apoptosis. As TGF-β signalling in CD8 + T cells is known to promote apoptosis of effector CD8 + T cells during the contraction phase [29] , [30] , we next monitored TGF-βRII expression at the surface of CD8 + T cells at different time points after LCMV infection ( Fig. 4f ). Consistent with their survival advantage, NK1.1 + CD8 + T cells maintained low levels of TGF-βRII at their surface, whereas TGF-βRII expression was gradually restored on NK1.1 − CD8 + T cells. Supporting their enhanced ability to escape apoptosis, at the peak of expansion (day 8), NK1.1 + CD8 + T had higher expression of the anti-apoptotic molecule Bcl-2 compared with NK1.1 − CD8 + T cells. In contrast, at 3 weeks post infection, immediately before the drop in NK1.1 + CD8 + T cell numbers ( Fig. 4a ), they expressed slightly lower Bcl-2 levels than NK1.1 − CD8 + T cells, which instead showed an increase in Bcl-2 levels ( Fig. 4g ). These data suggest that Bcl-2 dependent/TGF-β independent, late apoptosis of NK1.1 + CD8 + T cells may involve a defect in IL-2 and/or IL-15 sensitivity, as supported by the lower level of CD122 surface expression observed only on NK1.1 + CD8 + T cells in the third week following infection ( Fig. 4h ). Thus, this set of data reveals that, although the number of effector NK1.1 − CD8 + T cells rapidly decreases, the NK1.1 + CD8 + T-cell population remains constant for a longer period and accounts for a large proportion of pathogen-specific effector CD8 + T cells in the weeks following the NK1.1 − CD8 + T cell contraction. 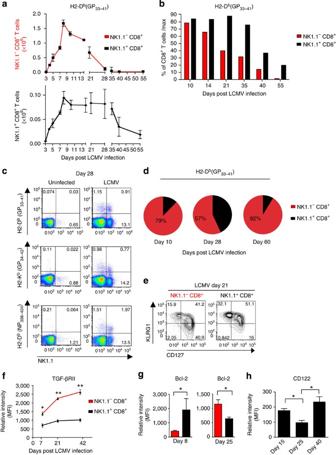Figure 4: NK1.1+CD8+T cells undergo a delayed contraction phase. (a) Graphs illustrating the absolute numbers of H2-Db(GP33–41) LCMV tetramer-specific CD8+T splenocytes at different times after B6 mice infection by LCMV. Data are representative of two independent experiments with three mice per point. (b) Histograms represent the percentage of H2-Db(GP33–41) CD8+T cells at different times after infection compared with their maximum at day 8 (100%). (c) Flow cytometry analysis of the proportion of several LCMV tetramer-specific NK1.1+and NK1.1−cells among CD8+splenocytes 28 days after LCMV infection. (d) Diagrams illustrate the repartition of H2-Db(GP33–41)-specific CD8+splenocytes in NK1.1+and NK1.1−cells at different times after LCMV infection. These results are representative of three independent experiments with two or three animals per group. (e) Flow cytometry analysis of the expression of KLRG1 and CD127 at the surface of H2-Db(GP33–41)-specific NK1.1+and NK1.1−CD8+T cells from the spleen 21 days after LCMV infection. (f,g) Mean of mean fluorescence intensity (MFI+s.d.) of the expression of TGF-βRII and Bcl-2 in H2-Db(GP33–41) LCMV-specific tetramer CD8+T splenocytes at different times after LCMV infection. (h) Graphs represent mean of MFI (+s.d.) of the expression of CD122 on H2-Db(GP33–41) LCMV-specific tetramer NK1.1+ CD8+T cells at different times after LCMV infection. These results are representative of two independent experiments with two or three animals per time point. Unpaired, two-tailed Student’st-test was used to assess the significance of differences observed between two groups.*P<0.05; **P<0.001. Figure 4: NK1.1 + CD8 + T cells undergo a delayed contraction phase. ( a ) Graphs illustrating the absolute numbers of H2-D b (GP 33–41 ) LCMV tetramer-specific CD8 + T splenocytes at different times after B6 mice infection by LCMV. Data are representative of two independent experiments with three mice per point. ( b ) Histograms represent the percentage of H2-D b (GP 33–41 ) CD8 + T cells at different times after infection compared with their maximum at day 8 (100%). ( c ) Flow cytometry analysis of the proportion of several LCMV tetramer-specific NK1.1 + and NK1.1 − cells among CD8 + splenocytes 28 days after LCMV infection. ( d ) Diagrams illustrate the repartition of H2-D b (GP 33–41 )-specific CD8 + splenocytes in NK1.1 + and NK1.1 − cells at different times after LCMV infection. These results are representative of three independent experiments with two or three animals per group. ( e ) Flow cytometry analysis of the expression of KLRG1 and CD127 at the surface of H2-D b (GP 33–41 )-specific NK1.1 + and NK1.1 − CD8 + T cells from the spleen 21 days after LCMV infection. ( f , g ) Mean of mean fluorescence intensity (MFI+s.d.) of the expression of TGF-βRII and Bcl-2 in H2-D b (GP 33–41 ) LCMV-specific tetramer CD8 + T splenocytes at different times after LCMV infection. ( h ) Graphs represent mean of MFI (+s.d.) of the expression of CD122 on H2-D b (GP 33–41 ) LCMV-specific tetramer NK1.1+ CD8 + T cells at different times after LCMV infection. These results are representative of two independent experiments with two or three animals per time point. Unpaired, two-tailed Student’s t -test was used to assess the significance of differences observed between two groups. *P <0.05; ** P <0.001. Full size image Interestingly, similar delayed contraction phase of NK1.1 + CD8 + T cells was also observed after Lm- Ova infection in mice previously transferred with OT-1 cells ( Supplementary Fig. 4 ) excluding a pathogen specificity of this phenomenon. We next took advantage of this OT-1 TCR transgenic model to monitor the individual outcome of both NK1.1 + CD8 + T cells and NK1.1 − CD8 + T cells. We first adoptively transferred congenic B6 mice by injection of OT-1 cells and subsequently infected them with Lm -Ova. Seven days later, NK1.1 + and NK1.1 − OT-1 cells were purified by flow-cell sorting and each population was separately transferred into Lm -Ova-infected matched congenic recipient mice reproducing the same infectious and inflammatory environment as that of cell-donor mice ( Fig. 5a ). Transferred cells were analysed on different days after infection. Notably, only a few % of the injected NK1.1 + CD8 + T cells had lost the NK1.1 marker at their surface and less than 5% of injected NK1.1 − CD8 + T cells expressed low levels of NK1.1, likely due to poor fidelity of cell sorting, ruling out a major inter-conversion between these two populations that could explain their changes of proportion during the evolving CD8 + T-cell response to infection ( Fig. 5b ). Given that coordinated expression of CD127 and KLRG1 has been proposed to distinguish short-lived effector cells (KLRG1 high , CD127 low ) from those destined to develop into memory T cells (KLRG1 − , CD127 high ) [1] , we then monitored the expression of these two markers at the surface of NK1.1 + CD8 + T cells and NK1.1 − CD8 + T cells ( Fig. 5c ). Both populations expressed mainly KLRG1 8 days after Lm -Ova infection, with a larger proportion of NK1.1 + CD8 + cells being KLRG1 high . In total agreement with our observations made during LCMV infection ( Figs 3a,b and 4e ), in contrast to the NK1.1 − CD8 + population that gradually lost KLRG1 high cells to be replaced by KLRG1 − CD127 high cells, we found that the NK1.1 + CD8 + cells remained KLRG1 high several weeks after Lm- Ova infection and gradually formed a KLRG1 CD127 double-positive population ( Fig. 5c ). As the loss of KLRG1 high CD8 + T cells (short-lived effector cells) was associated with an impairment of effector functions of the CD8 response in the weeks following the peak of the response [31] , we next assessed whether NK1.1 + CD8 + T cells maintained their effector functions several weeks after infection. Mice immunized as in Fig. 5a were re-challenged with Lm- Ova 2 weeks later. As expected, few NK1.1 − OT-1 cells were still able to produce both IFN-γ and granzyme B within 24 h in response to recall infection. In contrast, approximately 50% of the NK1.1 + OT-1 cells were still endowed with strong effector functions ( Fig. 5d,e ). It is notable that even among the KLRG1-positive cells, effector functions of NK1.1 − OT-1 T cells were largely impaired compared with that of KLRG1 + NK1.1 + OT-1 T cells ( Fig. 5f ). Thus, these results imply that NK1.1 + CD8 + T cells are long-lived effector cells and that they could sustain the control of potential novel pathogen intrusion by rapidly mounting effector function compared with their NK1.1 − counterparts. To further support this assumption, either NK1.1 + OT-1 cells or NK1.1 − OT-1 cells, purified from congenic B6 mice immunized with Lm -Ova 15 days prior, were separately grafted into B6 mice subsequently infected with Lm- Ova. One day later, we found a significantly reduced number of bacterial colony-forming units within the spleen of NK1.1 + OT-1 cell-grafted mice ( Fig. 5g ). Altogether, these results reveal NK1.1 + CD8 + T cells as a functionally distinct CD8 + population. Whereas NK1.1 − CD8 + T lymphocyte numbers and effector functions rapidly decreased after infection, the NK1.1 + CD8 + T-cell subset contracted substantially later and sustained prolonged effector functions and protection of the host, contributing to rapid anti-microbial CD8 + T-cell response. 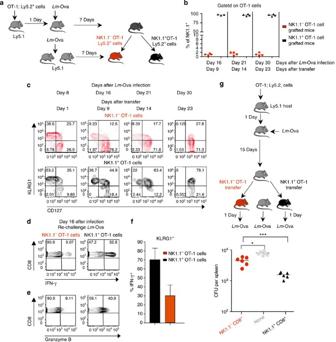Figure 5: NK1.1+CD8+T cells remain long-lived effector cells. (a) Illustration of the experimental procedure used to obtain data. For the first transfer, 500 OT-1 cells were grafted, and for the second, 105purified NK1.1+OT-1 and NK1.1−OT-1 cells were individually transferred in differentLm-Ova-infected matched congenic hosts. (b) Graph illustrates the percentage of NK1.1+cells among the OT-1 cells in the spleen of either NK1.1+OT-1 cell-grafted mice or NK1.1+OT-1 cell-grafted mice 9, 14 and 23 days after transfer. (c) Mice were analysed at different time points after infection for the co-expression of CD127 and KLRG1 on grafted cells. Data are representative of two experiments with three mice per each time point. (d–f) Host mice were re-challenged withLm-Ova at day 16 post infection and the ability of OT-1 cells to produce IFN-γ and granzyme B monitored 24 h later withoutin vitrore-stimulation. These results are representative of two experiments with two or three mice per group. (g) OT-1 cells were grafted in B6 mice infected the following day withLm-Ova. Fifteen days later, NK1.1+OT-1 cells and NK1.1−OT-1 cells were purified and 105cells separately transferred into B6 mice that were infected the following day byLm-Ova. The graph illustrates the colony-forming units (CFUs) observed per spleen 1 day after infection and is representative of three individual experiments. Unpaired, two-tailed Student’st-test was used to assess the significance of differences observed between two groups. *P<0.05; ***P<0.0001. Figure 5: NK1.1 + CD8 + T cells remain long-lived effector cells. ( a ) Illustration of the experimental procedure used to obtain data. For the first transfer, 500 OT-1 cells were grafted, and for the second, 10 5 purified NK1.1 + OT-1 and NK1.1 − OT-1 cells were individually transferred in different Lm -Ova-infected matched congenic hosts. ( b ) Graph illustrates the percentage of NK1.1 + cells among the OT-1 cells in the spleen of either NK1.1 + OT-1 cell-grafted mice or NK1.1 + OT-1 cell-grafted mice 9, 14 and 23 days after transfer. ( c ) Mice were analysed at different time points after infection for the co-expression of CD127 and KLRG1 on grafted cells. Data are representative of two experiments with three mice per each time point. ( d – f ) Host mice were re-challenged with Lm- Ova at day 16 post infection and the ability of OT-1 cells to produce IFN-γ and granzyme B monitored 24 h later without in vitro re-stimulation. These results are representative of two experiments with two or three mice per group. ( g ) OT-1 cells were grafted in B6 mice infected the following day with Lm -Ova. Fifteen days later, NK1.1 + OT-1 cells and NK1.1 − OT-1 cells were purified and 10 5 cells separately transferred into B6 mice that were infected the following day by Lm -Ova. The graph illustrates the colony-forming units (CFUs) observed per spleen 1 day after infection and is representative of three individual experiments. Unpaired, two-tailed Student’s t -test was used to assess the significance of differences observed between two groups. * P <0.05; *** P <0.0001. Full size image Memory NK1.1 + CD8 + T cells exhibit an effector-memory-like phenotype In humans and mice, NK1.1 + CD8 + T cells comprise 5–10% of the memory CD8 + T-cell population [19] . Interestingly, at the memory stage, we found that they sustained low levels of TGF-βRII expression and had the same tissue tropism as NK1.1 + CD8 + effector T cells ( Fig. 4e and Supplementary Figs 1 and 5 ). Surprisingly, 2 months after infection, KLRG1 CD127 double-positive cells were still largely prevalent (~60–70%) within the subset of memory NK1.1 + CD8 + T splenocytes, whereas they only represented a small fraction (~10–15%) of the memory NK1.1 − CD8 + T cells ( Fig. 6a ). Interestingly, a large proportion of NK1.1 + CD8 + memory T cells (~85%) were negative for the lymphoid organ homing molecule CD62L ( Fig. 6a ). As memory CD62L neg T cells have been associated with an effector-memory-like phenotype [32] , we next examined the capacity of the NK1.1 + CD8 + memory T cells to rapidly produce IFN-γ in response to cognate pathogen peptide ( Fig. 6b ). In contrast to their NK1.1 − counterparts, NK1.1 + CD8 + memory T cells specific for LCMV exhibited an exacerbated ability to rapidly produce IFN-γ after a short stimulation in vitro with cognate LCMV peptides, while maintaining their well-characterized difference of sensitivity between H2-D b (NP 396–404 )- and H2D b (GP 33–41 )-specific CD8 + T cells to their cognate antigen [33] ( Fig. 6b ). Thus, at the memory stage, NK1.1 + CD8 + T cells represent a distinct subset of memory CD8 + T cells that were mainly composed of KLRG1 CD127 double-positive cells, capable of quickly mounting an effective effector response to pathogen-derived antigens. 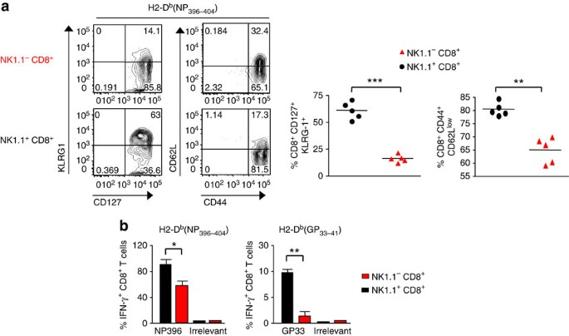Figure 6: NK1.1+CD8+T memory cells are effector memory-like T cells. B6 mice were infected with LCMV 66 days previously. (a) Mice were analysed by flow cytometry for the presence of H2-Db(NP396–404) tetramer+cells expressing NK1.1, KLRG1, CD127, CD44 and CD62L. (b) Graphs illustrate the mean of LCMV-specific tetramer+CD8+memory T cells producing IFN-γ 4 h afterin vitrore-stimulation with either cognate LCMV peptide (either NP396 or GP33) or irrelevant peptide (Ova). The mean of two experiments with two or three mice per groups (+s.d.) is illustrated. Unpaired, two-tailed Student'st-test was used to assess the significance of differences observed between two groups.*P<0.05; **P<0.001, ***P<0.0001. Figure 6: NK1.1 + CD8 + T memory cells are effector memory-like T cells. B6 mice were infected with LCMV 66 days previously. ( a ) Mice were analysed by flow cytometry for the presence of H2-D b (NP 396–404 ) tetramer + cells expressing NK1.1, KLRG1, CD127, CD44 and CD62L. ( b ) Graphs illustrate the mean of LCMV-specific tetramer + CD8 + memory T cells producing IFN-γ 4 h after in vitro re-stimulation with either cognate LCMV peptide (either NP396 or GP33) or irrelevant peptide (Ova). The mean of two experiments with two or three mice per groups (+s.d.) is illustrated. Unpaired, two-tailed Student's t -test was used to assess the significance of differences observed between two groups. * P <0.05; ** P <0.001, *** P <0.0001. Full size image NK1.1 + CD8 + memory T cells provide rapid innate immune protection Similar to NK cells, memory CD8 + T cells can be an early source of both IFN-γ and granzyme B in a cognate antigen-independent manner [13] , [14] , [34] , [35] . It is notable that NK1.1 + CD8 + memory T cells expressed surface makers associated with NK cells (data not shown). To address whether NK1.1 + CD8 + memory T cells were also endowed with functional characteristics of innate immune cells, mice previously infected with LCMV were subsequently challenged with Lm a few months later. IFN-γ production by memory LCMV-specific CD8 + T cells was then assessed in response to Lm infection ( Fig. 7a ). Remarkably, within a few hours after Lm injection, we observed approximately 50% more IFN-γ + cells among NK1.1 + CD8 + memory T cells compared with NK1.1 − counterparts. Moreover, these IFN-γ + NK1.1 + CD8 + memory T cells clearly expressed higher levels of IFN-γ ( Fig. 7a ). Similar observations were made in OT-1 memory cells generated in B6 mice grafted with OT-1 cells, primarily immunized with Lm -Ova and subsequently challenged with LCMV ( Fig. 7b,c ). Interestingly, a closer analysis of the kinetics revealed that NK1.1 + OT-1 memory splenocytes produced IFN-γ and granzyme B, both in larger frequency and more rapidly, compared with NK1.1 − OT-1 memory cells. In line with recent observations showing that early production of IFN-γ and granzyme B is orchestrated by IL-15 and IL-12 (refs 13 , 14 ), we observed that NK1.1 + CD8 + OT-1 memory cells were more sensitive to both IL-15 and IL-12 than their NK1.1 − counterparts ( Fig. 7d,e ). Thus, these data reveal that memory NK1.1 + CD8 + T cells are endowed with exacerbated innate-like features and respond earlier and more dramatically than their NK1.1 − counterparts to antigen nonspecific, cytokine-mediated stimulation, suggesting an important role for this memory cell-subset in the early control of pathogen propagation within the host. To confirm this assumption, LCMV-specific NK1.1 + or NK1.1 − CD8 + T cells were purified by flow-cell sorting from mice immunized with LCMV 60 days prior and adoptively transferred into naïve syngenic mice. Recipients were subsequently infected by Lm and their spleens analysed the next day to determine bacterial titres. We observed four- to fivefold reduction in bacterial colony-forming units in the spleen from mice grafted with LCMV-specific NK1.1 + CD8 + memory T cells compared with mice grafted with NK1.1 − cells ( Fig. 7f ). Altogether, these results support the idea that, among the memory CD8 + T cells, the NK1.1 + subset represents a unique subset that contributes efficiently to the early protective immune response against microbial pathogens. 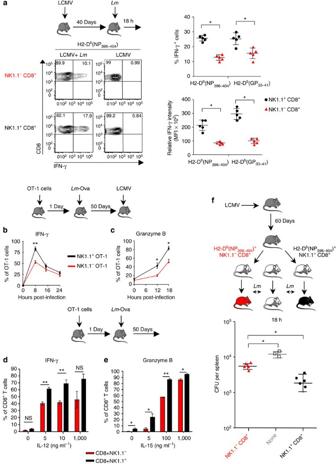Figure 7: Memory NK1.1+CD8+T cells produce rapidly IFN-γ and granzyme B in an innate-like manner. (a) Mice were infected with LCMV and subsequently re-infected or not 40 days later withLm. Percentages of H2-Db(NP396–404) tetramer-positive memory cells producing IFN-γ 14 h afterLminfection are represented. Graphs illustrate either the percentage of IFN-γ-positive memory cells or their mean fluorescence intensity in the spleen. (b,c) CD8+T cells from OT-1 Rag2KOwere grafted in B6 mice infected the following day withLm-Ova. Fifty days later, animals were infected with LCMV. The percentage OT-1 memory cells (H-2Kb(Ova) tetramers+) expressing IFN-γ and granzyme B at different hours post LCMV infection are illustrated by graph inaandc, respectively. Data are representative of two or three experiments with three to five animals per time points. (d,e) CD8+T cells from OT-1 Rag2KOwere grafted in B6 mice infected the following day withLm-Ova. Fifty days later, splenocytes were incubated with different concentrations of IL-15 and IL-12 for 12 h and the production of IFN-γ and granzyme B by H-2Kb(Ova) tetramer-positive CD8+T cells monitored by flow cytometry. Graph illustrates the mean of the percentage of IFN-γ and granzyme B (n=4+s.d.). (f) B6 mice were infected by LCMV 60 days earlier, H2-Db(NP396-404) tetramer-specific NK1.1+CD8+T cells and NK1.1−CD8+T cells were purified and separately grafted into B6 mice (5.103cells per recipient). Recipient animals were then infected the next day byLm. Graph illustratesLmtitration (colony-forming unit: CFU) in the spleens of different recipient animals 18 h later. Results are representative of two experiments with three or four animals per group. Unpaired, two-tailed Student’st-test was used to assess the significance of differences observed between two groups.*P<0.05; **P<0.001. NS, not significant. Figure 7: Memory NK1.1 + CD8 + T cells produce rapidly IFN-γ and granzyme B in an innate-like manner. ( a ) Mice were infected with LCMV and subsequently re-infected or not 40 days later with Lm . Percentages of H2-D b (NP 396–404 ) tetramer-positive memory cells producing IFN-γ 14 h after Lm infection are represented. Graphs illustrate either the percentage of IFN-γ-positive memory cells or their mean fluorescence intensity in the spleen. ( b , c ) CD8 + T cells from OT-1 Rag2 KO were grafted in B6 mice infected the following day with Lm -Ova. Fifty days later, animals were infected with LCMV. The percentage OT-1 memory cells (H-2K b (Ova) tetramers + ) expressing IFN-γ and granzyme B at different hours post LCMV infection are illustrated by graph in a and c , respectively. Data are representative of two or three experiments with three to five animals per time points. ( d , e ) CD8 + T cells from OT-1 Rag2 KO were grafted in B6 mice infected the following day with Lm -Ova. Fifty days later, splenocytes were incubated with different concentrations of IL-15 and IL-12 for 12 h and the production of IFN-γ and granzyme B by H-2K b (Ova) tetramer-positive CD8 + T cells monitored by flow cytometry. Graph illustrates the mean of the percentage of IFN-γ and granzyme B ( n =4+s.d.). ( f ) B6 mice were infected by LCMV 60 days earlier, H2-D b (NP 396-404 ) tetramer-specific NK1.1 + CD8 + T cells and NK1.1 − CD8 + T cells were purified and separately grafted into B6 mice (5.10 3 cells per recipient). Recipient animals were then infected the next day by Lm . Graph illustrates Lm titration (colony-forming unit: CFU) in the spleens of different recipient animals 18 h later. Results are representative of two experiments with three or four animals per group. Unpaired, two-tailed Student’s t -test was used to assess the significance of differences observed between two groups. *P <0.05; ** P <0.001. NS, not significant. Full size image After microbial pathogen invasion, one of the main challenges for the host is to rapidly control pathogen propagation to avoid vital tissue damage. Our results reveal that a unique subset of CD8 + T cells that express NK1.1 at their surface contribute to the early CD8 response to microbial recall infections, both at the effector and memory stage. In contrast with their NK1.1 − counterparts, for which both numbers and activity rapidly decrease after infection, the effector NK1.1 + CD8 + T cells are maintained longer and sustain prolonged microbiocidal activity. These long-lived effector cells ensure a rapid response to secondary microbial pathogen infections occurring during the period when pathogen-specific effector T cells are massively reduced and the memory CD8 response is not yet fully established [7] . Later, after undergoing contraction, NK1.1 + CD8 + T cells compose a pool of memory cells, expressing both KLRG-1 and CD127, endowed with exacerbated adaptive response and innate-like features, contributing again to the early control of microbial pathogen re-infections both in an antigen-dependent and -independent manner. It is well known that after infection, the expression levels of Tgfbr1 and Tgfbr2 complexes are rapidly downregulated after TCR engagement CD8 + T cells, either individually or together, to be gradually restored during the proliferation phase [36] . Our findings reveal that TGF-β represses differentiation of naïve NK1.1 − CD8 + T cells in NK1.1 + CD8 + T cells during infectious episodes, as CD8 + T cells that cannot control TGF-β signalling, fail to differentiate into NK1.1 + CD8 + T cells. Given that NK1.1 + CD8 + T cells were found in non-divided cells and KLRG1 − cells, we propose that their differentiation occurs during the initial priming-phase, likely before CD8 + T cells undergo significant expansion when Tgfbr expression is impaired [36] . NK1.1 + CD8 + T cells would merge from effector cells that maintain low levels of TGF-bR expression and sensitivity to TGF-β. It is possible that this specific differentiation, conditioned by the TGF-β signalling, is influenced by a dedicated cell localization within the spleen and regional cytokine microenvironment. Our work strongly suggests that the concerted action of inflammatory factors produced during infection, such as IL-15, is necessary for optimal CD8 + T-cell differentiation into NK1.1 + cells. However, like for numerous genes of klrg cluster, the expression klrb1c , encoding for NK1.1, seems dependent on STAT-5 but not directly regulated by this IL-15-activated transcription factors [37] . Although our results in vivo indicate that IL-15 signalling contributes to the downregulation of TGF-βR and enhances the NK1.1 expression at the surface of CD8 + T cells, they do not rule out additional suppressive effects of IL-15 signalling downstream of the TGF-β receptor, as suggested in T cells in vitro [27] , and the contribution of other inflammatory factors working in concert with IL-15. Whether NK1.1 + CD8 + T-cell differentiation occurs in the vicinity of cells selectively producing inflammatory cytokines in response to infection remains to be addressed. Interestingly, NK1.1 is a glycoprotein also expressed on NK cells and CD1d-dependent NKT cells, both lymphoid subsets that share several other NK surface markers and similar tissue tropism with NK1.1 + CD8 + T cells. It is notable that a similar dual role for IL-15 and TGF-β on NK1.1 expression has been also reported during the thymic development of CD1d-dependent NKT subsets [38] , [39] . Although the function of NK1.1 remains unclear, because of the absence of identified ligand in mice [19] , we do not exclude that NK1.1 expression by CD8 + T cells could reflect a differentiation stage of small numbers of pre-existing precursor cells, as for NK cells and CD1d-dependent NKT cells [38] , [39] . Such a hypothesis would explain why only a restricted proportion of TGF-βR low CD8 + T cells acquire the NK1.1 glycoprotein. As reported for NK cells NKT cells [40] , NK1.1 seems not having role in NK.1.1 + CD8 + T-cell development or function in vivo as, in Balb/c mice that contrary to humans and C57BL/6 mice do not expression NK.1.1 (CD161), CD8 + T cells expressing the other markers associated with NK.1.1 ( Supplementary figure 1 ) were still present and endowed with exacerbated effector functions ( Supplementary fig. 7 ). Like their NK1.1 − counterparts, NK1.1 + CD8 + T cells progress from effector cells to memory cells, however, we revealed that they behave on the fringes of the current paradigm. During a primary infection, it is well documented that most CD8 + T cells entering into effector end stage have a shortened lifespan and die following infection, while a smaller proportion of cells differentiate into memory cell precursors [1] . This longer survival of NK1.1 + CD8 + T cells is in agreement with previous gene expression analysis showing that klrb1c expression is enriched in pathogen-specific CD8 + T cells during the contraction phase [41] . Moreover, unlike certain effector cells, like Th17 (ref. 42 ), differentiated NK1.1 + CD8 + T cells seem stable at least under inflammatory conditions we analysed them. We propose that effector NK1.1 + CD8 + T cells fit into a unique differentiated CD8 + T-cell population with a longer effector lifespan accounted for by delayed contraction and sustained effector abilities. Notably, during both viral and bacterial infections, a wave of TGF-β production has been observed concomitantly to the beginning of the contraction phase [29] , [43] . TGF-β signalling in effector CD8 + T cells was reported as essential to promote their large-scale death by apoptosis, as CD8 + T cells expressing a dominant negative TGF-βRII survive much longer and maintain prolonged expression of high levels of Bcl-2 (ref. 29 ). We found that NK1.1 + CD8 + T cells maintain low surface levels of TGF-βR throughout their lifespan. Hence, in contrast to the majority of effector CD8 + T cells, they can control the pro-apoptotic effects of TGF-β and thus survive longer. This escape from apoptosis could explain why, several weeks after infection, effector NK1.1 + CD8 + T cells are still largely composed of KLRG1 high CD127 low cells, a population that has been reported with shortened life in many acute infections [1] . Although we do not rule out a role for other factors, such as IL-15 described to promote survival during the contraction phase [44] , the contribution of IL-15 in the delayed contraction of NK1.1 − CD8 + T cells is likely tenuous, as NK1.1 + CD8 + T effectors still contract later than their NK1.1 − counterparts in IL-15-deficient mice ( Supplementary Fig. 8 ). Thus, our results suggest that control of TGF-β sensitivity by programming TGF-βR expression might determine which antigen-specific CD8 + T cells may survive longer and prolong the anti-microbial response while the majority of the effector cells are dying. After contraction, and in contrast to NK1.1 − CD8 + T cells, NK1.1 + cells gradually accumulate as double-positive KLRG1 CD127 cells, a component of resting memory cells usually poorly represented among the bulk of memory CD8 + T cells. KLRG1 high CD127 high CD8 + memory T lymphocytes have been associated with cells that have experienced multiple infections by the same pathogen [45] , [46] . Although unlikely, we cannot exclude that NK1.1 + CD8 + T cells could interact with some antigen-presenting cells, sustaining prolonged pathogen-derived antigen presentation. We propose that, like NK1.1, the expression of KLRG1 is maintained at the surface of NK1.1 + CD8 + T cells throughout their lifespan. We reported that NK1.1 + CD8 + memory T cells can efficiently and rapidly mount an adaptive immune response against pathogen-derived antigens. Such functional ability could be explained by their diminished sensitivity to the well-characterized TGF-β-suppressive effects on both inflammatory and cytotoxic differentiation programmes [47] , [48] because of their sustained low expression of TGF-βR. Adaptive immune response of memory CD8 + T cells is considered to be a powerful response to re-infection, however, it only becomes fully efficient after a few days [8] , a delay during which pathogens could exploit weaknesses to progress in the organism. However, like NK cells, in response to a subsequent pathogen infection, memory CD8 + T cells have been described as producers of an early source of effector cytokines and cytotoxic molecules in a cognate antigen-independent manner [13] , [14] , [34] , [35] . This innate-like feature has recently been demonstrated to be induced in vivo through inflammasome activation, triggered by various microbial pathogen infections [14] . Memory CD8 + T cells are sensitive to inflammatory cytokines produced early by either dendritic cells [13] or inflammatory monocytes [14] . Even though they represent a small fraction of memory CD8 + T cells, we propose that memory NK1.1 + CD8 + T cells constitute a potent early line of defence against microbial pathogens by responding earlier and more efficiently than their NK1.1 − counterparts. Whether the expression of other NK-associated markers and their tissue tropism contribute to the ability of the memory NK1.1 + CD8 + T-cell subset to control early infection, remains to be addressed. In summary, our work revealed that, during infection, a part of primed T cells will escape from TGF-β signalling, by downregulating TGF-βR and can give rise to the NK1.1 + CD8 + T-cell subset. This unique population contributes to the early response to pathogen re-infection because of its prolonged microbiocidal activity by effector cells and its exacerbated innate-like features as memory T cells. Therefore, we propose that the NK1.1 + CD8 + subset complements the action of the arsenal of CD8 + T cells during early response against microbial pathogens as illustrated by Fig. 8 . Consequently, the development of vaccination adjuvants facilitating the differentiation of this subset will be of wide interest to speed up the control of pathogen propagation and thus to improve vaccine protection. 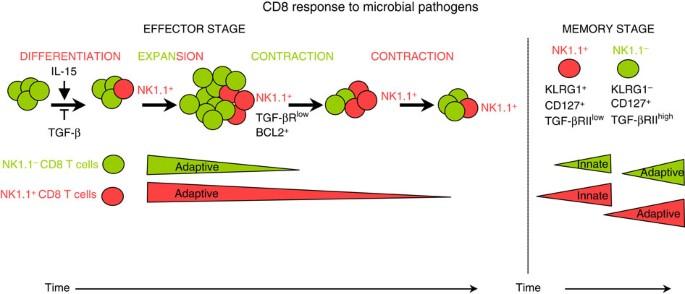Figure 8: Schematic overview of the difference between NK1.1–CD8+T cells and NK1.1+CD8+T cells responses to microbial pathogen. In response to microbial infection, a fraction of CD8+T cells can differentiate into NK1.1+CD8+T cells. This differentiation is blocked by TGF-β and enhanced by IL-15. Although NK1.1−cells, in green, rapidly contract and loss their adaptive effector function, cells that acquire the NK1.1 marker, in red, contract much later and sustain longer effector functions and host protection. At the memory stage, NK1.1+cells respond rapidly and strongly to pathogen in an innate-like manner, and develop more rapid and efficient adaptive memory response than their CD8+memory T-cell counterparts. Figure 8: Schematic overview of the difference between NK1.1 – CD8 + T cells and NK1.1 + CD8 + T cells responses to microbial pathogen. In response to microbial infection, a fraction of CD8 + T cells can differentiate into NK1.1 + CD8 + T cells. This differentiation is blocked by TGF-β and enhanced by IL-15. Although NK1.1 − cells, in green, rapidly contract and loss their adaptive effector function, cells that acquire the NK1.1 marker, in red, contract much later and sustain longer effector functions and host protection. At the memory stage, NK1.1 + cells respond rapidly and strongly to pathogen in an innate-like manner, and develop more rapid and efficient adaptive memory response than their CD8 + memory T-cell counterparts. Full size image Mice C57BL/6 (B6) mice, B6 Thy.1.1 congenic mice, Balb-c, OT-1 and Rag2 KO mice were purchased from Charles-Rivers. B6 CD4-Cre; Stop fl/fl Tgf- β RI CA transgenic animals were generated as previously described [24] . IL-15 KO mice were purchased from Taconic. Tomato-OT-1 mice were generated as previously described [14] . CD1d KO mice were provided by Dr L.Van Kaer (Vanderbilt University, Nasville, TN). Mice were maintained in a specific pathogen-free animal facility at the ‘Plateau de Biologie Experimental de la Souris (PBES)’ (Lyon, France) and AniCan centre Léon Bérard (Lyon, France) or SPF animal facility Albert Einstein College of Medicine (AECOM). Six- to eight–week-old female mice were used at the beginning of the experiments. Animal experiments were carried out in strict accordance with the recommendations by the Animal Use Committees CECCAPP (Comité d'Evaluation Commun au PBES, à AniCan, au laboratoire P4) at the Cancer Research Center of Lyon and at the AECOM. Viral and bacterial infections and peptide immunization LCMV Armstrong was kindly provided by Dr R. Ahmed (Atlanta, USA) and amplified in BHK-21 cells as described [49] . 2 × 10 5 plaque-forming units of Armstrong strain were injected i.p. for acute infection. Both Lm 10403s and Lm -Ova, expressing Ovalbumin (Ova) peptide, were provided by Dr H. Shen. Bacteria were adapted to mice as described [29] . 2,000–5,000 bacteria were injected i.v. Bacterial titration was performed from spleen extract on Brain Heart Infusion soft agar (Fluka). Peptide immunization was performed by 2 intra-peritoneal injections over two subsequent days with 50 nM of Ova (SIINFEKL; NeoMPS) diluted in PBS (Invitrogen). Lymphocyte isolation, purification and transfer Cell suspensions were prepared from the spleen, liver, thymus, blood and peripheral lymph nodes as described previously [47] . CD8 + T cells were purified using anti-CD8-conjugated magnetic beads (Miltenyi). Enriched CD8 + T cell fraction was then stained for NK1.1 + and CD8 + as well as for CD44-, CD62L- or LCMV-specific tetramers or Thy1.2 when indicated and sorted using a two laser BD FACS Aria (BD Biosciences) cell sorter/analyser. 500–1,000 of purified naïve OT-1 cells were transferred i.v. into mice. Antibodies and flow cytometry Anti-mouse Bcl-2, BrdU (3D4), CD4 (GK1.5), CD5 (53 7.3) CD8 (53-6.7), NK1.1 (PK136), CD44 (IM-7), CD62L (MEL-14), CD90.1 (HIS51), CD90.2 (53-2.1), CD94 (18d3), CD127 (A7R34), CD107, DX5 (DX5), NKG2A/C/E (20d5) NKG2D (C7), IFN-γ (XMG 1.2), KLRG1 (2F1), LY49C/I/F Ly6C (AL-21), TCR-β (H57-597) and TNF-α (MP6-XT22) and streptavidine were purchased from BD Biosciences or eBioscience. Anti-mouse TGF-βRII (BAF532), used at one-tenth, was purchased from R&D Systems and anti-human granzyme B (GB11) was purchased from Invitrogen. Intracellular and intranuclear staining were performed using Cytofix/Cytoperm (BD Biosciences) and FoxP3 staining buffer kit (ebioscience), respectively, according to the provider’s guidelines. For cytokine staining, when indicated, splenocytes were incubated with LCMV NP396 (FQPQNGQFI) peptide or with LCMV GP33 (KAVYNFATC) (NeoMPS) for 4 h, in the presence of 1 μg ml −1 Golgi Plug (BD Biosciences). LCMV iTAg MHC Tetramer NP396 (FQPQNGQFI) Allele H-2 D b /PE, iTAg MHC Tetramer GP33 (KAVYNFATC) Allele H-2D b /PE GP34/PE and Ova iTag Tetramer Ova (SIINFEKL) Allele H-2K b /PE were purchased from Beckman Coulter and provided by the NIH tetramer facility. Flow cytometry analysis was carried out on Canto II and Fortessa cytometers (BD Biosciences). When it is not mentioned antibodies were used at 1/200. BM chimeras BM cells from Thy1.1 C57BL/6 mice and Thy1.2 C57BL/6 CD4-Cre; Stop fl/fl TGF-bRI CA mice were isolated and depleted of CD3 + cells using anti-CD3 beads (Miltenyi-Biotec). One million cells of each genotype were mixed (1:1) and transferred intravenously into irradiated Rag2 KO recipient mice (8 Gray). Mice were infected 6 weeks after transfer by LCMV Armstrong. BrdU administration BrdU (Sigma) was given to animals in their drinking water 0.8 mg ml −1 at the time infection and for 8 further days. In vitro culture Splenocytes were incubated for 14 h at 37 °C in the presence of either mouse recombinant IL-15 (R&D Systems) or mouse recombinant IL-12 (PeproTech) in RPMI (10% foetal calf serum, 2 mM L -glutamine, 100 U l −1 penicillin/streptomycin, 1 mM HEPES) with Golgi Plug (BD Biosciences). TCR repertoire Purified DNA from NK1.1 + CD8 + T cells was analysed for Vβ chain diversity (Immun ID). Statistics Unpaired, two-tailed Student’s t -test were used to assess the significance of differences observed between two groups with GraphPad Prism software. P values are given as: * P <0.05; ** P <0.001, *** P <0.0001. How to cite this article: Ruiz, A. L. et al. NK1.1 + CD8 + T cells escape TGF-β control and contribute to early microbial pathogen response. Nat. Commun. 5:5150 doi: 10.1038/ncomms6150 (2014).